Microbiome remodelling leads to inhibition of intestinal farnesoid X receptor signalling and decreased obesity The antioxidant tempol reduces obesity in mice. Here we show that tempol alters the gut microbiome by preferentially reducing the genus Lactobacillus and its bile salt hydrolase (BSH) activity leading to the accumulation of intestinal tauro-β-muricholic acid (T-β-MCA). T-β-MCA is an farnesoid X receptor (FXR) nuclear receptor antagonist, which is involved in the regulation of bile acid, lipid and glucose metabolism. Its increased levels during tempol treatment inhibit FXR signalling in the intestine. High-fat diet-fed intestine-specific Fxr -null ( Fxr ΔIE ) mice show lower diet-induced obesity, similar to tempol-treated wild-type mice. Further, tempol treatment does not decrease weight gain in Fxr ΔIE mice, suggesting that the intestinal FXR mediates the anti-obesity effects of tempol. These studies demonstrate a biochemical link between the microbiome, nuclear receptor signalling and metabolic disorders, and suggest that inhibition of FXR in the intestine could be a target for anti-obesity drugs. Obesity has reached epidemic proportions worldwide and is associated with chronic diseases such as type 2 diabetes mellitus, cardiovascular diseases, hepatosteatosis and cancer [1] . Obesity develops as a result of energy intake that exceeds energy expenditure, thus leading to a net storage of excess calories in the form of fat in adipose tissue [2] . Thus, a pharmaceutical approach that suppresses appetite, blocks dietary fat absorption or promotes fat mobilization would be ideal [3] . Tempol (4-hydroxy-2,2,6,6-tetramethylpiperidine 1-oxyl), an antioxidant and a radiation protector [4] , [5] , was reported to prevent obesity in mice [6] . A recent mass spectrometry-based metabolomic investigation revealed that tempol altered levels of suspected gut microbe-generated metabolites, thus providing initial clues that tempol may either change the composition of the microbiome or alter the metabolic potential of gut bacteria [7] . Interestingly, tempol can also inhibit the harmful effects of ischaemia/reperfusion injury on intestinal tissues of rats through its prevention of bacterial translocation [8] . However, the influence of tempol on the gut microbiome has not been explored. High-throughput 16S ribosomal RNA (16S rRNA) gene sequencing of gut microbial populations and mass spectrometry-based metabolomics are powerful tools for characterization of the gut microbiome and metabolites in biological matrices, respectively [9] , [10] . It is known that disruption of the gut microbiome balance in the intestine can affect different metabolic pathways in vivo such as fatty-acid and bile-acid metabolism [11] . This may contribute to the findings that the phylum Firmicutes and the phylum Bacteroidetes, the two predominant populations of microbiota in both mice and humans, are altered in obese mice as compared with lean animals [12] . It was predicted that the marriage of 16S rRNA sequencing, metagenomics and metabolomics could shed light on the interaction between the host and the 100 trillion microbes residing in the gut [13] . However, to date, there have been limited studies using these high-throughput approaches with respect to the identification of potential targets for treating obesity and insulin resistance. In the current study, a combination of 16S rRNA gene sequencing and mass spectrometry-based metabolomics was adopted to investigate changes in the gut microbiome and metabolites in a high-fat diet (HFD)-fed mouse model undergoing tempol treatment. Further, intestine-specific Fxr -null ( Fxr ΔIE ) mice were employed to explore the mechanism by which the gut microbiome influences obesity and insulin resistance. This study demonstrates that tempol decreases obesity and insulin resistance by remodelling the intestinal microbiota, leading to a change in the composition of bile acids and associated inhibition of farnesoid X receptor (FXR) signalling. Tempol protects mice from obesity and insulin resistance Tempol is a member of a family of nitroxide compounds that promotes the metabolism of many reactive oxygen species. Although tempol was found to reduce body weight gain, the exact mechanism was unclear. Tempol treatment reduces body weight gain after 3 weeks of treatment with a HFD ( Supplementary Fig. S1a ). Body composition, measured by nuclear magnetic resonance (NMR), confirms that the fat mass, fat/body mass ratios and fat/lean mass ratios in tempol-treated mice are decreased significantly after 16 weeks of tempol treatment compared with vehicle-treated mice ( Supplementary Figs S1b,S2a ). Food and water intake is comparable between the two groups ( Supplementary Fig. S2b–c ). To explore the role of tempol in obesity-related glucose homoeostasis, glucose and insulin tolerance tests (GTT and ITT) were performed. GTT reveals that after 11 weeks of HFD challenge, tempol-treated mice display significantly reduced blood glucose levels after glucose loading compared with vehicle-treated mice ( Supplementary Fig. S1c ). ITT demonstrate that the insulin sensitivity is significantly increased in tempol-treated mice ( Supplementary Fig. S1d ). Moreover, fasted serum insulin levels show a decreased trend and the calculated homoeostasis model assessment measurement of insulin resistance is significantly lower in tempol-treated mice ( Supplementary Fig. S1e ). These results confirm that tempol improved HFD-induced insulin resistance, which may be due in large part to the decrease in adiposity. Tempol affects gut microbiota and BSH activity Earlier studies indicated that tempol increased the urinary excretion of 2,8-dihydroxyquinoline and its glucuronide metabolites that are generated by bacteria residing in the gut [14] , [15] . These observations suggested that tempol might affect gut microbial metabolism or the composition of the gut microbiome. Indeed, significant phylum-level shifts from Firmicutes to Bacteroidetes in the gut microbiome composition are observed in mouse caecum following 5 days of tempol administered by gavage (250 mg kg −1 per day) to mice on a normal chow diet ( Fig. 1a ). Heat map diagrams of 16S rRNA sequencing results indicate that tempol treatment dramatically decreases the family Lactobacillaceae ( Fig. 1b ) and robustly reduces the genus Lactobacillus ( Fig. 1c ). Similar to the results of acute treatment via gavage, quantitative real-time PCR (qPCR) analysis of suspected caecum microbes obtained from mice on a HFD reveals that tempol treatment causes a shift from Firmicutes to Bacteroidetes ( Fig. 1d ). These results indicate that the effects of tempol on the gut microbiome are independent of diet, delivery method, and obesity. Further, the genus Lactobacillus of the Lactobacillaceae is decreased, coincident with a significantly lower bile salt hydrolase (BSH) enzymatic activity in the feces ( Fig. 1e ). BSH deconjugates taurine-conjugated bile acids produced in the liver to free bile acids [16] . In addition, the genus Clostridium was also reported to be involved in bile-acid metabolism, including deconjugation, 7-dehydroxylation, oxidation and epimerization. The major secondary bile acids are deoxycholic acid (DCA) and murideoxycholic acid, which are the 7-dehydroxylation products of cholic acid and β-muricholic acid (β-MCA), respectively [17] . Tempol treatment also decreases levels of the genus Clostridium cluster IV and Clostridium cluster XIVa ( Supplementary Fig. S3 ) that were reportedly increased in obesity [18] . These results suggest that tempol remodelling of the gut microbiome contributes to altered bile-acid metabolism. 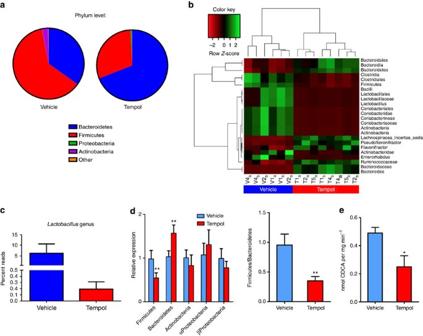Figure 1: Tempol treatment induces gut micriobiome robust shifts. (a) 16S rRNA gene sequencing analysis at the phylum levels of caecum content after 5 days of tempol treatment by gavage (250 mg kg−1).n=3 per vehicle group,n=4 per tempol group. (b) The heat map of 16S rRNA gene sequencing analysis of caecum content after 5 days of tempol treatment by gavage (250 mg kg−1). The scale: green colours indicate high values, whereas red colours indicate low values for the percent of reads that were classified at that rank. (c) 16S rRNA gene sequencing analysis of genusLactobacilluscaecum content after 5 days of tempol treatment by gavage (250 mg kg−1).n=3 per vehicle group,n=4 per tempol group. Data are presented as mean±s.d. (d) qPCR analysis of phylum-level modifications from 16S rRNA of fecal microbiome after tempol treatment on a HFD for 12 weeks.n=5 mice per group. Data are presented as mean±s.d., ANOVA followed by two-tailed Student’st-test. **P<0.01 compared with vehicle-treated mice. (e) Fecal BSH enzyme activity on vehicle- and tempol-treated mice on a HFD for 12 weeks.n=5 mice per group. All data are presented as mean±s.d., ANOVA followed by two-tailed Student’st-test. *P<0.05, **P<0.01 compared with vehicle-treated mice. Figure 1: Tempol treatment induces gut micriobiome robust shifts. ( a ) 16S rRNA gene sequencing analysis at the phylum levels of caecum content after 5 days of tempol treatment by gavage (250 mg kg −1 ). n =3 per vehicle group, n =4 per tempol group. ( b ) The heat map of 16S rRNA gene sequencing analysis of caecum content after 5 days of tempol treatment by gavage (250 mg kg −1 ). The scale: green colours indicate high values, whereas red colours indicate low values for the percent of reads that were classified at that rank. ( c ) 16S rRNA gene sequencing analysis of genus Lactobacillus caecum content after 5 days of tempol treatment by gavage (250 mg kg −1 ). n =3 per vehicle group, n =4 per tempol group. Data are presented as mean±s.d. ( d ) qPCR analysis of phylum-level modifications from 16S rRNA of fecal microbiome after tempol treatment on a HFD for 12 weeks. n =5 mice per group. Data are presented as mean±s.d., ANOVA followed by two-tailed Student’s t -test. ** P <0.01 compared with vehicle-treated mice. ( e ) Fecal BSH enzyme activity on vehicle- and tempol-treated mice on a HFD for 12 weeks. n =5 mice per group. All data are presented as mean±s.d., ANOVA followed by two-tailed Student’s t -test. * P <0.05, ** P <0.01 compared with vehicle-treated mice. Full size image Tempol enhances the intestinal taurine-conjugated bile acids Previous studies demonstrated that alteration of the gut microbiome affects the levels of bile acids in the liver, heart and kidney [19] . To determine whether the composition of bile acids were changed in the tempol group, ultra-performance liquid chromatography coupled with electrospray ionization quadrupole time-of-flight mass spectrometry (UPLC-ESI-QTOFMS)-based metabolomics analysis was used to examine the bile-acid composition and their levels in the feces and intestinal tissue. Partial least-squares discriminant analysis (PLS-DA) modelling of the UPLC-ESI-QTOFMS-negative mode data from mouse feces and intestine reveal distinct clustering of the control and tempol groups ( Supplementary Fig. S4 ). Levels of the four ions ( m/z , 453.2842 at 3.14 min; m/z , 391.2841 at 4.11 min; m/z , 407.2782 at 3.33 min; and m/z , 391.2838 at 4.06 min) are significantly reduced in the feces by tempol ( Fig. 2a ), whereas four ions ( m/z , 514.2864 at 2.53 min; m/z , 514.2862 at 2.91 min; m/z , 498.2910 at 2.85 min; and m/z , 498.2891 at 3.22 min) are markedly enriched in the intestine of tempol-treated mice ( Fig. 2b ). Ion identification was performed by tandem mass spectrometry and retention time comparisons with authentic standards ( Supplementary Figs S5,S6 ). The attenuated four ions are identified as four free bile acids, namely β-MCA, DCA, γ-muricholic acid (γ-MCA) and chenodeoxycholic acid (CDCA). In contrast to feces, the four increased ions in the intestine are taurine-conjugated bile acids, tauro-β-muricholic acid (T-β-MCA), taurocholic acid (TCA), tauroursodeoxycholic acid (TUDCA) and taurochenodeoxycholic acid (TCDCA). The most significantly enriched bile acid is T-β-MCA in the PLS-DA scatter plot. Metabolomics results were further verified by direct bile-acid analysis indicating that the total bile acids are reduced in the feces but increased in the intestine by tempol ( Fig. 2c,d ). Further, the individual bile-acid composition in feces and the intestine was examined between the control and tempol-treated groups revealing that tempol decreases most free bile-acid species in the feces and increases taurine-conjugated bile acid levels in the intestine ( Fig. 2e,f ). Intestinal TCA, T-β-MCA and TCDCA is increased 5.4-fold, 8.8-fold and 3.1-fold by tempol treatment, respectively ( Fig. 2f ). 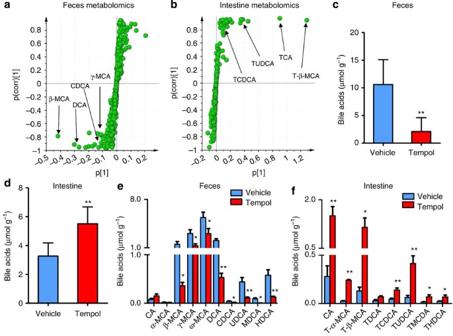Figure 2: Metabolomics analysis identifies the alteration of bile-acid composition by tempol. (a) Scatter plot of PLS-DA of fecal ions from vehicle and tempol treatment in HFD-fed mice. Each point represents an individual mouse fecal ion. The labelled ions were identified as β-MCA, DCA, CDCA and γ-MCA, which were decreased by tempol treatment. The p(corr)[1]P-values represent the interclass difference and p[1]P-values represent the relative abundance of the ions. All data were obtained in negative mode (ESI−). (b) Scatter plot of PLS-DA of intestinal ions from vehicle and tempol treatment on a HFD-fed mice. Each point represents an individual mouse intestinal ion. The labelled ions are identified to be T-β-MCA, TCA, TUDCA and TCDCA, which were increased by tempol treatment. The p(corr)[1] values represent the interclass difference and p[1] values represent the relative abundance of the ions. All data are obtained in negative mode (ESI−). (c) Total level of bile acid in feces of the vehicle and tempol group on a HFD for 12 weeks.n=5 mice per group. (d) Total level of bile acid in the intestine of vehicle and tempol group on a HFD for 17 weeks.n=5 mice per group. (e) Bile-acid composition in feces of the vehicle and tempol group on a HFD for 12 weeks.n=5 mice per group. (f) Bile-acid composition in the intestine of vehicle and tempol group on a HFD for 17 weeks.n=5 mice per group. The total bile acids were quantified by bile-acid kit and bile-acid composition was determined using UPLC-ESI-QTOFMS. All data are presented as mean±s.d., ANOVA followed by two-tailed Student’st-test. *P<0.05, **P<0.01 compared with vehicle-treated mice. Figure 2: Metabolomics analysis identifies the alteration of bile-acid composition by tempol. ( a ) Scatter plot of PLS-DA of fecal ions from vehicle and tempol treatment in HFD-fed mice. Each point represents an individual mouse fecal ion. The labelled ions were identified as β-MCA, DCA, CDCA and γ-MCA, which were decreased by tempol treatment. The p(corr)[1] P -values represent the interclass difference and p[1] P -values represent the relative abundance of the ions. All data were obtained in negative mode (ESI−). ( b ) Scatter plot of PLS-DA of intestinal ions from vehicle and tempol treatment on a HFD-fed mice. Each point represents an individual mouse intestinal ion. The labelled ions are identified to be T-β-MCA, TCA, TUDCA and TCDCA, which were increased by tempol treatment. The p(corr)[1] values represent the interclass difference and p[1] values represent the relative abundance of the ions. All data are obtained in negative mode (ESI−). ( c ) Total level of bile acid in feces of the vehicle and tempol group on a HFD for 12 weeks. n =5 mice per group. ( d ) Total level of bile acid in the intestine of vehicle and tempol group on a HFD for 17 weeks. n =5 mice per group. ( e ) Bile-acid composition in feces of the vehicle and tempol group on a HFD for 12 weeks. n =5 mice per group. ( f ) Bile-acid composition in the intestine of vehicle and tempol group on a HFD for 17 weeks. n =5 mice per group. The total bile acids were quantified by bile-acid kit and bile-acid composition was determined using UPLC-ESI-QTOFMS. All data are presented as mean±s.d., ANOVA followed by two-tailed Student’s t -test. * P <0.05, ** P <0.01 compared with vehicle-treated mice. Full size image T-β-MCA inhibits the FXR signalling pathway Bile-acid metabolism is tightly associated with the FXR signalling pathway, and HFD can induce FXR signalling in the intestine [20] . Tempol treatment inhibits expression of the FXR target genes small heterodimer partner ( Shp ), fibroblast growth factor 15 ( Fgf15 ) and intestinal bile acid-binding protein, indicating that FXR signalling is markedly decreased in the small intestine ( Fig. 3a ). FXR signalling is not altered in the liver of tempol-treated mice ( Fig. 3b ). In addition, Shp expression is not decreased in HepG2 cells after 200 μM tempol exposure at baseline and after co-treatment of cells with tempol and the FXR agonist 100 μM CDCA ( Supplementary Fig. S7 ). These results indicate that tempol indirectly inhibits the FXR signalling pathway. Tempol treatment also increases the levels of several taurine-conjugated bile acids (T-β-MCA, TCA, TCDCA and TUDCA) in the intestine. Thus, the question arose as to whether specific taurine-conjugated bile acids can inhibit the FXR signalling pathway. In vitro , 100 μM TCA increases Shp mRNA expression by 2.5-fold, whereas the induction of Shp mRNA with 100 μM TCDCA is 1.7-fold, 100 μM TUDCA has no effect and 100 μM T-β-MCA inhibits Shp expression in primary mouse hepatocytes ( Fig. 3c ). More importantly, 100 μM T-β-MCA and TCDCA significantly inhibits Shp mRNA expression after exposure of cells to 100 μM TCA ( Fig. 3d ). To further demonstrate the inhibition of FXR by T-β-MCA in the intestine, the human intestinal cell line CaCo2 was transfected with a luciferase construct driven by an FXR control element. Luciferase assays demonstrate that T-β-MCA antagonizes FXR activation by TCA ( Fig. 3e ). These results provide compelling evidence that T-β-MCA is an endogenous antagonist of FXR in the intestine, which can inhibit basal FXR signalling and TCA-activated signalling, consistent with a previous report showing inhibition of FXR activation by T-β-MCA in vitro and in vivo [21] . TCDCA can also inhibit FXR signalling after TCA exposure. These data further suggest that the inhibition of FXR signalling in the intestine by tempol treatment is mainly due to the accumulation of intestinal T-β-MCA. 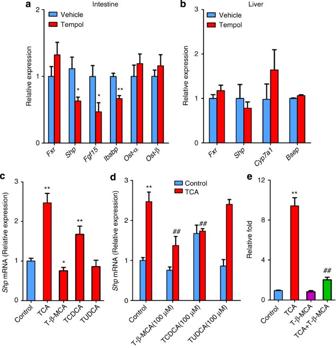Figure 3: T-β-MCA inhibits the FXR signalling pathway. (a) mRNA levels of FXR target genes in the intestine on vehicle- and tempol-treated mice on a HFD. Expression was normalized to 18S RNA.n=5 mice per group. All data are presented as mean±s.d., ANOVA followed by two-tailed Student’st-test.*P<0.05, **P<0.01 compared with vehicle-treated mice. (b) mRNA levels of FXR target genes in the liver on vehicle- and tempol-treated mice on a HFD. Expression was normalized to 18S RNA.n=5 mice per group. Data are presented as mean±s.d., ANOVA followed by two-tailed Student’st-test. *P<0.05, **P<0.01 compared with vehicle-treated mice. (c)ShpmRNA expression of primary hepatocytes after treatment with 100 μM TCA, T-β-MCA, TCDCA and TUDCA (n=4). Expression was normalized to 18S RNA. All data are presented as mean±s.d., ANOVA followed by two-tailed Student’st-test. *P<0.05, **P<0.01 compared with control. (d)ShpmRNA expression of primary hepatocytes after exposure to 100 μM T-β-MCA, TCDCA or TUDCA with 100 μM TCA (n=4). Expression was normalized to 18S RNA. All data are presented as mean±s.d., ANOVA followed by one-way ANOVA with Dunnett’s test. **P<0.01 compared with control,##P<0.01 compared with TCA (100 μM) treatment. (e) Luciferase assays of the inhibition of FXR by T-β-MCA in CaCo2 cells. CaCo2 cells are transfected with a PGL4-Shp-TK firefly luciferase construct, the control plasmid phRL-SV40, human FXR and human ASBT expression plasmids. After 24 h, the cells are treated with 100 μM TCA, T-β-MCA or T-β-MCA with 100 μM TCA.n=4. All data are presented as mean±s.d., ANOVA followed by one-way ANOVA with Dunnett’s test. **P<0.01 compared with control,##P<0.01 compared with TCA treatment. Figure 3: T-β-MCA inhibits the FXR signalling pathway. ( a ) mRNA levels of FXR target genes in the intestine on vehicle- and tempol-treated mice on a HFD. Expression was normalized to 18S RNA. n =5 mice per group. All data are presented as mean±s.d., ANOVA followed by two-tailed Student’s t -test. *P <0.05, ** P <0.01 compared with vehicle-treated mice. ( b ) mRNA levels of FXR target genes in the liver on vehicle- and tempol-treated mice on a HFD. Expression was normalized to 18S RNA. n =5 mice per group. Data are presented as mean±s.d., ANOVA followed by two-tailed Student’s t -test. * P <0.05, ** P <0.01 compared with vehicle-treated mice. ( c ) Shp mRNA expression of primary hepatocytes after treatment with 100 μM TCA, T-β-MCA, TCDCA and TUDCA ( n =4). Expression was normalized to 18S RNA. All data are presented as mean±s.d., ANOVA followed by two-tailed Student’s t -test. * P <0.05, ** P <0.01 compared with control. ( d ) Shp mRNA expression of primary hepatocytes after exposure to 100 μM T-β-MCA, TCDCA or TUDCA with 100 μM TCA ( n =4). Expression was normalized to 18S RNA. All data are presented as mean±s.d., ANOVA followed by one-way ANOVA with Dunnett’s test. ** P <0.01 compared with control, ## P <0.01 compared with TCA (100 μM) treatment. ( e ) Luciferase assays of the inhibition of FXR by T-β-MCA in CaCo2 cells. CaCo2 cells are transfected with a PGL4- Shp -TK firefly luciferase construct, the control plasmid phRL-SV40, human FXR and human ASBT expression plasmids. After 24 h, the cells are treated with 100 μM TCA, T-β-MCA or T-β-MCA with 100 μM TCA. n =4. All data are presented as mean±s.d., ANOVA followed by one-way ANOVA with Dunnett’s test. ** P <0.01 compared with control, ## P <0.01 compared with TCA treatment. Full size image Intestine-specific FXR disruption reduces obesity To further explore the role of intestinal FXR in lipid and glucose metabolism, male wild-type ( Fxr fl/fl ) mice and intestine-specific Fxr -null ( Fxr ΔIE ) mice were fed a HFD, revealing that the body weights of Fxr ΔIE mice are lower than Fxr fl/fl mice after 3 weeks of treatment ( Fig. 4a ). NMR measurements confirm that the fat mass, the ratio of fat and body mass and the ratio of fat and lean mass of Fxr fl/fl mice on a HFD are higher than Fxr ΔIE mice ( Fig. 4b , Supplementary Fig. S8a ). Food intake measurements are comparable between Fxr fl/fl and Fxr ΔIE mice ( Supplementary Fig. S8b ). GTT reveals that Fxr ΔIE mice have improved glucose intolerance compared with Fxr fl/fl mice ( Fig. 4c ) and ITT demonstrates that the insulin sensitivity in Fxr ΔIE mice is significantly increased ( Fig. 4d ). Moreover, fasted serum insulin levels and the homoeostasis model assessment index are significantly reduced in Fxr ΔIE mice ( Fig. 4e ). The expression of Fxr mRNA is nearly absent in the intestinal mucosa of Fxr ΔIE mice and, accordingly, expression of the FXR target genes Fgf15 , organic solute transporter-α and organic solute transporter-β are significantly lower ( Supplementary Fig. S8c ). In particular, the fatty-acid trafficking-related genes encoding fatty-acid-binding protein 4 and fatty-acid-binding protein 6 are markedly decreased, whereas expression of genes involved in fatty acid β-oxidation such as peroxisome proliferator-activated receptor-α, carnitine palmitoyltransferase 2, acyl-Coenzyme A oxidase 1, acyl-Coenzyme A oxidase 2 and acyl-CoA synthetase long-chain family member 1 are elevated ( Fig. 5a,b ). 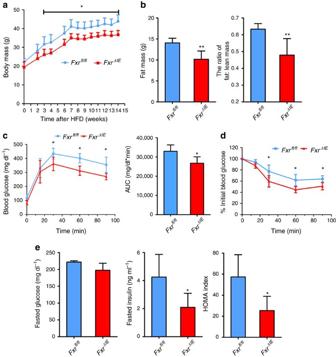Figure 4: Intestine-specific FXR knockout mice are resistant to obesity and insulin resistance. (a) Typical growth curves of the mice maintained on a HFD.n=5 mice per group. (b) The fat mass and fat mass to lean mass ratio of the mice on 6 weeks of HFD.n=5 mice per group. (c) GTT and the area under the curve on 7 weeks of HFD.n=5 mice per group. (d) ITT on 13 weeks of HFD.n=5 mice per group. (e) Fasted glucose, fasted serum insulin levels and homoeostasis model assessment index on 14 weeks of HFD.n=5 mice per group. All data are presented as mean±s.d., ANOVA followed by two-tailed Student’st-test. *P<0.05, **P<0.01 compared withFxrfl/flmice. Figure 4: Intestine-specific FXR knockout mice are resistant to obesity and insulin resistance. ( a ) Typical growth curves of the mice maintained on a HFD. n =5 mice per group. ( b ) The fat mass and fat mass to lean mass ratio of the mice on 6 weeks of HFD. n =5 mice per group. ( c ) GTT and the area under the curve on 7 weeks of HFD. n =5 mice per group. ( d ) ITT on 13 weeks of HFD. n =5 mice per group. ( e ) Fasted glucose, fasted serum insulin levels and homoeostasis model assessment index on 14 weeks of HFD. n =5 mice per group. All data are presented as mean±s.d., ANOVA followed by two-tailed Student’s t -test. * P <0.05, ** P <0.01 compared with Fxr fl/fl mice. 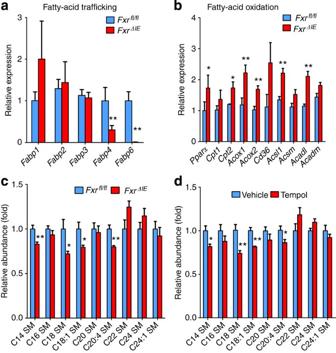Figure 5: Intestine-specific FXR deletion increases lipid oxidation and decreases serum sphingolipids. (a) qPCR analysis of fatty-acid trafficking-related genes in the intestinal mucosa ofFxrfl/flmice andFxrΔIEmice on a HFD for 14 weeks. Expression was normalized to 18S.n=5 mice per group. (b) qPCR analysis of fatty-acid trafficking- and mobilization-related genes in the intestinal mucosa ofFxrfl/flmice andFxrΔIEmice on a HFD for 14 weeks. Expression was normalized to 18S RNA.n=5 mice per group. (c) Lipidomics profile of serum sphingomyelin (SM) ofFxrfl/flmice andFxrΔIEmice on a HFD for 14 weeks. All data are presented as mean±s.d., ANOVA followed by two-tailed Student’st-test. *P<0.05, **P<0.01 compared withFxrfl/flmice. (d) Lipidomics profile of serum SM after tempol treatment on a HFD for 17 weeks.n=5 mice per group. Data are presented as mean±s.d., ANOVA followed by two-tailed Student’st-test. *P<0.05, **P<0.01 compared with vehicle-treated mice. Full size image Figure 5: Intestine-specific FXR deletion increases lipid oxidation and decreases serum sphingolipids. ( a ) qPCR analysis of fatty-acid trafficking-related genes in the intestinal mucosa of Fxr fl/fl mice and Fxr ΔIE mice on a HFD for 14 weeks. Expression was normalized to 18S. n =5 mice per group. ( b ) qPCR analysis of fatty-acid trafficking- and mobilization-related genes in the intestinal mucosa of Fxr fl/fl mice and Fxr ΔIE mice on a HFD for 14 weeks. Expression was normalized to 18S RNA. n =5 mice per group. ( c ) Lipidomics profile of serum sphingomyelin (SM) of Fxr fl/fl mice and Fxr ΔIE mice on a HFD for 14 weeks. All data are presented as mean±s.d., ANOVA followed by two-tailed Student’s t -test. * P <0.05, ** P <0.01 compared with Fxr fl/fl mice. ( d ) Lipidomics profile of serum SM after tempol treatment on a HFD for 17 weeks. n =5 mice per group. Data are presented as mean±s.d., ANOVA followed by two-tailed Student’s t -test. * P <0.05, ** P <0.01 compared with vehicle-treated mice. Full size image Earlier studies revealed that C14, C18, C18:1, C20:4 sphingomyelins (SMs) and ceramide to sphingosine-1-phosphate ratios were positively correlated with insulin resistance [22] , [23] . Serum lipidomics using tandem mass spectrometry and retention time comparisons with ion identification and quantification with authentic standards ( Supplementary Fig. S9a,b ), reveals that these compounds are decreased in both Fxr ΔIE mice ( Fig. 5c , Supplementary Fig. S9c ) and tempol-treated mice ( Fig. 5d , Supplementary Fig. S9c ), thus further indicating that inhibition of intestinal FXR may contribute to tempol-mediated improvement of HFD-induced metabolic dysfunction. Tempol improves obesity via inhibition of intestinal FXR To further investigate the role of FXR in the tempol-improved metabolic phenotype of HFD-fed mice, wild-type ( Fxr +/+ ) mice and whole-body Fxr -null ( Fxr −/− ) mice, wild-type ( Fxr fl/fl ) mice and intestine-specific Fxr -null ( Fxr ΔIE ) mice on a HFD were administered tempol in the drinking water. The body mass of tempol-treated Fxr +/+ and Fxr fl/fl mice are significantly decreased, respectively, whereas in Fxr −/− and Fxr ΔIE mice, body masses are comparable between vehicle and tempol-treated mice ( Fig. 6a , Supplementary Fig. S10a ). Body compositions confirmed that tempol decreases fat mass and fat/lean mass ratios in Fxr fl/fl mice but not in Fxr ΔIE mice ( Fig. 6b ). GTT further indicates that tempol improved glucose intolerance in Fxr +/+ and Fxr fl/fl mice, respectively, whereas no improvement is noted in Fxr −/− and Fxr ΔIE mice treated with tempol ( Fig. 6c , Supplementary Fig. S10b ). In addition, ITT analysis reveals that tempol ameliorate insulin sensitivity in Fxr +/+ mice but not in Fxr −/− mice ( Fig. 6d , Supplementary Fig. S10c ). Tempol treatment decreases fasted serum glucose, insulin levels and the HOMA index in Fxr fl/fl mice, whereas no improvement is noted in Fxr ΔIE mice treated with tempol ( Fig. 6e ). Previous studies reported that the total bile-acid pool size was increased in Fxr −/− mice, with no significant difference noted in the pool size between wild-type and Fxr ΔIE mice [24] . However, the levels of T-β-MCA and other taurine-conjugated bile acids are increased in the intestine of Fxr fl/fl and Fxr ΔIE mice following tempol treatment ( Supplementary Fig. S11 ), thus suggesting that the increased T-β-MCA results from the altered gut microbiota composition following tempol treatment, and not from the inhibition of intestinal FXR. The present findings reveal that inhibition of intestinal FXR is a major contributing factor for tempol to improve HFD-induced metabolic dysfunction. 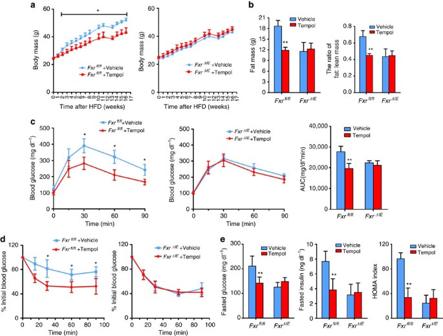Figure 6: The inhibition of intestinal FXR is crucial for tempol to improve metabolic profile. (a) Growth curves of vehicle- and tempol-treatedFxrfl/flmice andFxrΔIEmice on a HFD.n=4-5 mice per group. (b) Body composition by NMR to show the fat mass (left) and fat mass to lean mass ratio (right) in vehicle- and tempol-treated mice on 13 weeks of HFD.n=4–5 mice per group. (c) GTT and the area under the curve after 5 weeks of tempol-treated mice on a HFD.n=4–5 mice per group. (d) ITT after 6 weeks of HFD.n=4–5 mice per group. (e) Fasted glucose, fasted serum insulin levels and homoeostasis model assessment index after tempol treatment on a HFD for 16 weeks.n=5 mice per group. All data are presented as mean±s.d., ANOVA followed by one-way ANOVA with Tukey’s test. *P<0.05, **P<0.01 compared with vehicle-treated mice of the same genotype. Figure 6: The inhibition of intestinal FXR is crucial for tempol to improve metabolic profile. ( a ) Growth curves of vehicle- and tempol-treated Fxr fl/fl mice and Fxr ΔIE mice on a HFD. n =4-5 mice per group. ( b ) Body composition by NMR to show the fat mass (left) and fat mass to lean mass ratio (right) in vehicle- and tempol-treated mice on 13 weeks of HFD. n =4–5 mice per group. ( c ) GTT and the area under the curve after 5 weeks of tempol-treated mice on a HFD. n =4–5 mice per group. ( d ) ITT after 6 weeks of HFD. n =4–5 mice per group. ( e ) Fasted glucose, fasted serum insulin levels and homoeostasis model assessment index after tempol treatment on a HFD for 16 weeks. n =5 mice per group. All data are presented as mean±s.d., ANOVA followed by one-way ANOVA with Tukey’s test. * P <0.05, ** P <0.01 compared with vehicle-treated mice of the same genotype. Full size image The current study demonstrated that tempol improves obesity and insulin resistance via inhibition of the intestinal FXR. It is likely that the increase in insulin sensitivity after tempol treatment is attributed to the decrease of obesity. The combination of two high-throughput methods, 16S rRNA gene sequencing of the gut microbiome and metabolomics, were adopted to examine changes in the gut microbiota and metabolites in mice following tempol treatment, respectively. Within the intestinal microbiome, at the phylum level, tempol treatment profoundly shifted the microbial community from Firmicutes towards Bacteroidetes. The genus Lactobacillus in the phylum Firmicutes was almost completely abolished in the caecum of tempol-treated mice compared with the control group. The changes in the microbiome after tempol administration are in agreement with a recent study implicating changes in the gut bacteria population based on changes in urinary metabolites known to be derived from the gut flora [7] . In a rat model of superior mesenteric artery occlusion, tempol treatment prevented the harmful effects of ischaemia/reperfusion injury on intestinal tissues by reducing bacterial translocation [8] . These results provide further evidence that tempol can affect the microbiome. The effects of tempol on the gut microbiome and obesity are in agreement with earlier studies, which demonstrated that the gut microbiome can affect nutrient absorption and energy regulation [25] . Metagenomics analysis also indicated that the composition of gut microbiome in feces and caecum was different between obese and lean animals and humans, in particular, and in agreement with the present study, Firmucutes are more prevalent in obese humans and mice than in their lean counterparts [12] . The phylum Firmicutes, which has a role in the generation of butyrate, formate and lactate, represents about 50% of the total gut microbiome in the body [10] . Recently, several reports indicated an association between Lactobacillaceae and the development of obesity [26] . Here the population of Lactobacillus was decreased after tempol treatment, which is consistent with studies showing that Lactobacillus populations are elevated in obese and diabetic subjects [27] and decreased after gastric bypass surgery [28] , one of the most effective treatments for severe obesity. Metabolomics analysis revealed that the levels of taurine-conjugated bile acids were increased in the intestine of the tempol-treated group, probably a direct result of lower BSH activity from Lactobacillus . Indeed, among the Firmucutes, members of the genus Lactobacillus have BSH activity and carry out deconjugation of taurine-conjugated bile acids in the intestine [29] . In the tempol-treated group, the lower bile salt hydrolase activity, which converts T-β-MCA to MCA, probably contributed to the accumulation of T-β-MCA. Interestingly, T-β-MCA was found to be a novel antagonist of FXR in this work and an earlier study [21] . TCDCA, a weak agonist of FXR, can also inhibit FXR activation by another FXR agonist, such as TCA. This suggests that in the present study, the FXR signalling pathway is significantly inhibited in the tempol group as a result of increased T-β-MCA and TCDCA in the intestine. In agreement with the current study, the level of taurine-conjugated bile acids was elevated in germ-free mice that show a lean phenotype compared with normal mice [19] , [30] . The fact that HFD-fed Fxr ΔIE mice have a similar metabolic phenotype as mice under tempol treatment and they did not exhibit increased weight loss as compared with vehicle-treated HFD-fed Fxr ΔIE mice thus indicates a central role for FXR in tempol efficacy. Although the anti-obesity effect of tempol is correlated with alteration of the gut microbiome composition and is in agreement with other correlative metagenomic studies in mice and humans, it should be noted that earlier studies proposed that tempol decreases obesity by lowering reactive oxygen species and leptin secretion from adipose tissue [31] . However, in the present work, it is unlikely that tempol has major antioxidant effects in this target tissue because of the very low drug concentration in the intestine obtained by oral administration. A recent study revealed that the gut microbiota regulates host body energy homoeostasis via the short-chain fatty-acid receptor GPR43-G(i/o)βγ-PLC–PKC–PTEN pathway [32] . The potential role of GPR43 signalling pathway in the effect of tempol on obesity requires further experimentation. In any case, although it cannot be ruled out that tempol has other effects that also have an impact on obesity, the current findings provide evidence that gut microbiota and intestinal FXR signalling have a major influence on tempol-improved obesity. FXR has a key role in bile acid, lipid and glucose metabolism. Fxr −/− mice had increased glucose intolerance on a chow diet [33] and FXR agonists improved insulin sensitivity in a genetic mouse model of obesity [34] . However, other studies indicated that Fxr −/− mice had improved glucose homoeostasis and that FXR agonist aggravated disorders in lipid metabolism and insulin resistance in obese mouse models [35] , [36] . This contradictory evidence on the role of FXR in the pathogenesis of metabolic disorders might be because of signalling by the FXR in the liver in contrast to the present study implicating intestinal FXR. In addition, differences in the gut microbiota could explain the discrepant experimental results previously reported. In the current study, evidence is presented to support the view that the inhibition of intestinal FXR in both the genetic ablation Fxr ΔIE mouse model and in tempol-treated mice ameliorate diet-induced obesity and insulin resistance. Although the full mechanism of how intestinal FXR signalling influences obesity is not fully established, lipidomics revealed that serum C14, C18, C18:1, C20:4 SM and the ceramide to S1P ratios are decreased in both Fxr ΔIE mice and tempol-treated mice. In the last decade, numerous studies support a role for SM and its metabolites in the pathogenesis of obesity-associated metabolic disorders [22] . SM can be metabolized to ceramide, sphingosine and S1P [37] . Ceramide activates protein kinase C, c-Jun N-terminal kinase and inhibits the transmission of the insulin signalling pathway in peripheral insulin target tissues such as the liver and adipose tissue [38] . S1P was reported to counteract the effects of ceramide. It was shown that increased ceramide to S1P ratio contributes to insulin resistance and obesity [39] . Whether this is a major pathway mediating the effects of tempol and FXR on obesity, warrants further investigation. In summary, metagenomics and metabolomics revealed that inhibition of intestinal FXR signalling by tempol treatment was associated with decreased Lactobacillus and its BSH activity. The accumulation of T-β-MCA in the intestine was accompanied by inhibition of FXR. A recent study revealed by use of germ-free mice that T-β-MCA could inhibit FXR signalling in vivo in the intestine [21] . This is in support of the in vitro studies reported herein. The finding that tempol improved obesity via inhibition of intestinal FXR signalling suggests that intestinal FXR could act as a potential clinical target for the treatment of obesity. Chemicals and reagents Tempol was purchased from Sigma (St. Louis, MO). Bile acids were ordered from Steraloid, Inc. (Newport, RI) and Sigma, and TCA-d5 sodium salt was from Toronto Research Chemicals Inc. (Toronto, Ontario). SMs and ceramides were obtained from Avanti Polar Lipids. The S1P ELISA kit was purchased from Echelon Biosciences Inc. (Salt Lake City, UT). The bile acid kit was purchased from Catachem, Inc. (Oxford, CT). All solvents and organic reagents were of the highest grade available. Animal studies The wild-type ( Fxr +/+ ) mice and whole-body Fxr -null ( Fxr −/− ) mice, and, wild-type ( Fxr fl/fl ) mice and intestine-specific Fxr -null ( Fxr ΔIE ) mice are all on a C57BL/6N genetic background [24] , [40] . Fxr +/+ and Fxr −/− [40] mice were backcrossed with C57BL/6N mice for over four generations. Fxr fl/fl and Fxr ΔIE [24] mice were backcrossed with C57BL/6N mice for over 10 generations. The mice were housed in temperature- and light-controlled rooms and given water and pelleted NIH-31 chow ad libitum . All animal studies were performed in accordance with Institute of Laboratory Animal Resources guidelines and approved by the National Cancer Institute Animal Care and Use Committee. In the tempol study, male mice were fed a HFD (Bio-Serv, Frenchtown, NJ; 60 kcal% fat) from 6 weeks of age and administered 0.064% (w/v) tempol in the drinking water. For the chow diet study, tempol (dissolved in 0.9% normal saline) was orally administered to C57BL/6N mice for 5 days [7] . When food and water intakes were measured, the mice were removed from their home cage and transferred to a metabolic cage and housed individually. The mice were adapted to the metabolic cages for 1 day, and the cumulative food and water intakes were then measured for 5 days. A single mouse was placed in a single metabolic cage and five mice per group were analysed. Twenty-four-hour feces were collected from mice housed individually in metabolic cages (Jencons, Leighton Buzzard, UK). Body composition was measured in mice using an Echo3-in-1 NMR analyser (Echo Medical Systems, Houston, TX). Blood samples were collected by retro-orbital bleeding at the end of tempol treatment. Liver, intestine and caecum samples were collected immediately following killing by CO 2 asphyxiation. All samples were stored at −80 °C until analysis. Preparation and culture of primary hepatocytes Hepatocytes were prepared by the general perfusion method [41] . Primary hepatocytes from 6-week-old C57BL/6N mice were obtained by collagenase 1 (Invitrogen, Carlsbad, CA) perfusion. The cells were purified by 45% percoll (Sigma-Aldrich, St Louis, MO) density centrifugation and cultured in DMEM (Invitrogen) with 10% fetal bovine serum and 1% insulin-transferrin-selenium-ethanolamine (Invitrogen). The viability of hepatocytes was determined using trypan blue dye exclusion and those with higher than 85% viability were used. The medium was changed to DMEM with 1% fetal bovine serum after culturing for 4 h. After starvation for 4 h, the cells were exposed to tempol/TCA/T-β-MCA/TCDCA/ TUDCA/CDCA for 24 h. RNA analysis The mucosa of intestine was gently scraped and flash frozen in liquid nitrogen and stored at −80 °C until RNA was prepared. RNA was extracted from frozen intestine using TRIzol reagent (Invitrogen). Complementary DNA was synthesized from 1 μg of total RNA using Superscript II reverse transcriptase (Invitrogen). qPCR primers were designed with qPrimerDepot and the sequences are shown in the Supplementary Table S1 . qPCR was carried out using SYBR green PCR master mix in an ABI Prism 7900HT sequence detection system (Applied Biosystems, Foster City, CA). Measured mRNA levels were normalized to those of 18S ribosomal RNA and expressed as fold change relative to those of control group. Luciferase assays Grace Guo (Rutgers University) provided the PGL4-Shp-TK firefly luciferase construct and human Fxr expression plasmid. Paul A. Dawson (Wake Forest University School of Medicine) provided human Asbt expression plasmid. The plasmids were transfected into Caco2 (ATCC HTB-37) cells using the X-tremeGENE HP DNA Transfection Reagent (Roche Diagnostics, Indianapolis, IN). The cells were lysed and luciferase activities were measured with a Dual-Luciferase assay kit (Promega, Madison, WI). Firefly luciferase activity was normalized to Renilla luciferase activity. Metabolic assays For GTT, mice were fasted for 16 h, blood was drawn and mice were injected intraperitoneally with 1 g kg −1 glucose. For ITT, mice were fasted for 4 h, blood was drawn and then injected intraperitoneally with insulin (Eli Lilly, Washington, DC) 1 U kg −1 body weight. Blood samples were taken from the tail at 15, 30, 60 and 90 min after injection, and glucose was measured using a glucometer (Bayer, Pittsburgh, PA). Fasted serum insulin was measured using an enzyme-linked immunosorbent assay kit (Crystal Chem Inc., Downers Grove, IL). 16S rRNA gene sequencing of the intestinal microbiome The bacteria in feces and caecum content were extracted using PowerSoil DNA Isolation Kit (Mo Bio laboratory, Inc., Carlsbad, CA). The PCR products (~1,000 bp) were purified using the AgencourtAMPure technology (Beckman Coulter, Brea, CA) as described in 454 Technical Bulletin number 2011-002, Short Fragment Removal Procedure. After purification, the products were quantified by both Qubit (Lifetech, Carlsbad, CA) and qPCR, using the KAPA Biosystems Library Quantification Kit (KapaBiosystems, Woburn, MA). Products were pooled based on molar amounts, run on a 1% agarose gel and extracted. After clean-up with a QIAquick PCR Purification kit (Qiagen, Valencia, CA), quality and quantity were assessed using a DNA 7500LabChip on the Agilent 2100 Bioanalyzer (Agilent Technologies, Santa Clara, CA) and Qubit quantification. The sequencing was performed using a quarter Picotiter Plate on a 454 Life Sciences Genome Sequencer FLX+ (Roche Diagnostics). qPCR was carried out using SYBR green PCR master mix in an ABI Prism 7900HT sequence detection system (Applied Biosystems). PCR conditions were 50 °C for 2 min; 95 °C for 10 min; 40 cycles of 95 °C for 15S; and 60 °C for 1 min. Metagenomic data analysis The experimental set-up consisted of 14 samples distributed as 6 vehicle replicates and 8 tempol gavage replicates. After quality filtering and deduplication, each sample contains on average 11,000 reads. The mothur software package [42] was used to preprocess the sequencing data and the Ribosomal Database Project multi-classifier [43] to assign each sequence to a taxonomic rank. Preprocessing consisted of filtering reads for an average quality of 20, removing duplicated sequences and splitting into samples by barcodes, while allowing for one mismatch in the barcode. A custom statistical tool using analysis of variance (ANOVA) with factorial treatment design detects taxonomic ranks that show statistically significant changes between the samples. To account for differences in total reads per sample, classifications were converted to percent of total reads. This approach then permitted accurate comparisons within and between groups. ANOVA analysis with factorial treatment design was introduced to detect bacteria that significantly changed in numbers. The full model is called the fixed effects model. Treatments tempol and vehicle Study: study 1, study 2 (re-sequencing of study 1) Hypothesis: bacteria are unchanged under different doses. Full model: with i =1, 2, 3; j =1, 2; k =1, 2, 3, 4 Reduced model: with i =1, 2, 3; k =1, 2, 3, 4 The full model treats the two studies (study 1 and study 2) as a block to first see whether there is a ‘study’ effect. If the ‘study’ effect is significant, the studies are kept separate in the problem as a block effect [42] . If not, it is removed and combined with data from two studies [43] . Finally, the Šidák correction was employed for P -value correction. UPLC-ESI-QTOFMS analysis UPLC-ESI-QTOFMS analysis was performed in positive and negative mode, which was operated in full-scan mode at m/z 100–1,000 (ref. 44 ). The liquid chromatography system was an ACQUITY UPLC (Waters Corp., Milford, MA) consisting of a reverse-phase 2.1 × 50 mm ACQUITY UPLC BEH C18 1.7 μm column (Waters Corp.) with a gradient mobile phase comprising 0.1% formic-acid solution (A) and acetonitrile containing 0.1% formic-acid solution (B). The gradient was maintained at 100% A for 0.5 min, increased to 100% B over the next 7.5 min and returned to 100% A in last 2 min. Nitrogen was used as both cone gas (50 l h −1 ) and desolvation gas(600 l h −1 ). Source temperature and desolvation temperature were set at 120 °C and 350 °C, respectively. The capillary voltage and cone voltage were 3,000 and 20 V, respectively. Quantitation of bile-acid composition was determined using UPLC-ESI-QTOFMS. Quantitation of ceramides in serum, fecal and intestinal sample was performed using an ACQUITY UPLC system coupled with a XEVO triple quadrupole tandem mass spectrometer (Waters Corp.). The concentration of metabolites was quantified by multiple reaction-monitoring mass spectrometry based on standard curves using authentic standards. Fecal samples were prepared by adding 20 mg of feces to 400 μl of phosphate-buffered saline, homogenized and centrifuged at 18,000 × g for 20 min. The intestinal tissues were removed and flushed with ice-cold phosphate-buffered saline. The intestine was cut open longitudinally and the mucosa was gently scraped off and flash frozen in liquid nitrogen. Intestinal samples (20 mg) were extracted with 20-fold 50% acetonitrile, homogenized and centrifuged at 18,000 × g for 20 min. The homogenate was diluted with nine volumes of 66% acetonitrile and centrifuged at 18,000 × g for 20 min. Serum lipids were extracted from serum samples (25 μl) using four-volume chloroform/methanol (2:1). After centrifugation at 18,000 × g for 20 min, the organic phase was evaporated under a N2 stream. The lipid extract was dissolved in 25 μl chloroform/methanol (1:1) and diluted to a final solution with 10-volume isopropanol/acetonitrile/water (50/25/25). To identify the metabolites with high-contribution score in the S-plot, metabolomics databases (METLIN and Madison Metabolomics Consortium Database) were searched to find potential candidates. To confirm the identities of the putative markers, authentic standards were compared with the metabolites in the serum, fecal and intestinal sample based on MS/MS fragmentation pattern and retention time. Data processing and multivariate data analysis Raw data were aligned using MarkerLynx software (Waters Corp.) to generate a data matrix consisting of peak areas corresponding to a unique m/z and retention time without normalization. Metabolomics analysis including principal component analysis and PLS-DA models was performed with SIMCA-P+12 (Umetrics, Kinnelon, NJ) [44] . The ions with a correlation of ⩾ 0.8 to the model significantly contributed to the separation between control group and tempol-treated group. BSH activity Fecal proteins were prepared from the fecal sample (0.5 g) in pH 7.4 PBS (5.0 ml) using sonication [45] . BSH activity was measured based on the generation of CDCA from TCDCA in the feces. Briefly, incubation was carried out in 3 mM sodium acetate buffer, pH 5.2, containing 0.1 mg ml −1 fecal protein and 50 μM TCDCA-d5 in a final volume of 200 μl. After a 20-min incubation at 37 °C, the reaction was stopped by plunging the samples into dry ice. One hundred microlitres of methanol were directly added to the 100-μl reaction mix. After centrifuging at 14,000 × g for 20 min, 5 μl of the supernatant was transferred to an auto sampler vial subjected to analysis by a UPLC system coupled with a XEVO triple quadrupole tandem mass spectrometer (Waters Corp.). Data analysis Experimental values are presented as mean±s.d., statistical analysis were performed using the two-tailed Student’s t -test and the one-way ANOVA with Tukey’s test and Dunnett’s test, respectively. P -values<0.05 were considered significant. How to cite this article: Li, F. et al. Microbiome remodelling leads to inhibition of intestinal farnesoid X-receptor signalling and decreased obesity. Nat. Commun. 4:2384 doi: 10.1038/ncomms3384 (2013).